Solid-state electronic spin coherence time approaching one second Solid-state spin systems such as nitrogen-vacancy colour centres in diamond are promising for applications of quantum information, sensing and metrology. However, a key challenge for such solid-state systems is to realize a spin coherence time that is much longer than the time for quantum spin manipulation protocols. Here we demonstrate an improvement of more than two orders of magnitude in the spin coherence time ( T 2 ) of nitrogen-vacancy centres compared with previous measurements: T 2 ≈0.6 s at 77 K. We employed dynamical decoupling pulse sequences to suppress nitrogen-vacancy spin decoherence, and found that T 2 is limited to approximately half of the longitudinal spin relaxation time over a wide range of temperatures, which we attribute to phonon-induced decoherence. Our results apply to ensembles of nitrogen-vacancy spins, and thus could advance quantum sensing, enable squeezing and many-body entanglement, and open a path to simulating driven, interaction-dominated quantum many-body Hamiltonians. In recent years, the electronic spin of the negatively charged nitrogen-vacancy (NV) colour centre in diamond has become a leading platform for applications ranging from quantum information processing [1] to quantum sensing and metrology [2] , [3] , [4] . Importantly, the NV spin-state can be optically initialized and detected on a timescale of ~300 ns ( [5] ) and coherently driven at up to gigahertz rates [5] . Single NV centres in isotopically engineered high-purity diamond can possess long electronic spin coherence times on the order of a few millisecond at room temperature [6] . By applying dynamical decoupling sequences, similar coherence times can be achieved for single NV centres [7] , [8] , [9] and NV ensembles [10] in diamond containing higher impurity concentration. Here we apply dynamical decoupling techniques to ensembles of NV centres over a range of temperatures (77 K–300 K) in order to suppress both decoherence [10] and phononic spin relaxation [11] . We demonstrate an extension of the NV spin coherence time ( T 2 ) to T 2 ≈0.6 s at 77 K, which corresponds to an improvement of more than two orders of magnitude compared with previous measurements [6] , [10] and is on par with the longest coherence times achieved for electronic spins in any solid-state system [12] . Over a wide range of temperatures we also find that the NV spin T 2 is limited to approximately half of the longitudinal spin relaxation time ( T 1 ), T 2 ≈0.5 T 1 , a finding that could be relevant to other solid-state spin defects (such as P donors in Si). The present result of NV T 2 approaching 1 s, in combination with single NV optical addressability and the practicality and scalability of diamond, advance NV centres to the forefront of candidates for quantum information, simulation and sensing applications [1] , [2] . Coherence decay and longitudinal relaxation As an example of our data, we plot in Fig. 1 the measured NV spin coherence as a function of time for Carr-Purcell-Meiboom-Gill (CPMG) pulse sequences [13] with different numbers of pulses n , at room temperature T =300 K (a) and at T =160 K (b), for an isotopically pure (0.01% 13 C) diamond sample with nitrogen density ~10 15 cm −3 and NV density ~3 × 10 12 cm −3 (see Methods section for details). For each of these decoherence curves, we extracted T 2 by fitting the data to a stretched exponential function , where the p parameter is related to the dynamics of the spin environment and inhomogeneous broadening due to ensemble averaging [14] . For both temperatures T 2 increases with the number of pulses in the CPMG sequence and is limited to about half of T 1 : at 300 K, T 2 =3.3(4) ms and T 1 =6.0(4) ms; and at 160 K, T 2 =40(8) ms and T 1 =77(5) ms. 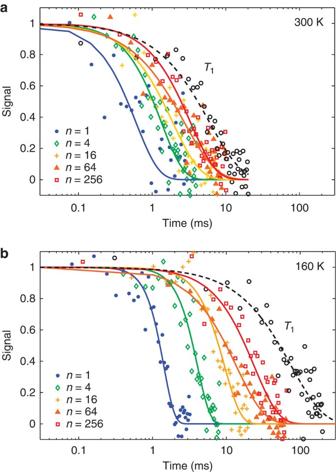Figure 1: Measured coherence decay and longitudinal relaxation. Measured NV spin coherence decay used to determineT2forn-pulse CPMG sequences (coloured data points and solid line fits to data), and longitudinal spin relaxation used to determineT1(black data points and dashed line fits to data), at (a)T=300 K and (b)T=160 K. Figure 1: Measured coherence decay and longitudinal relaxation. 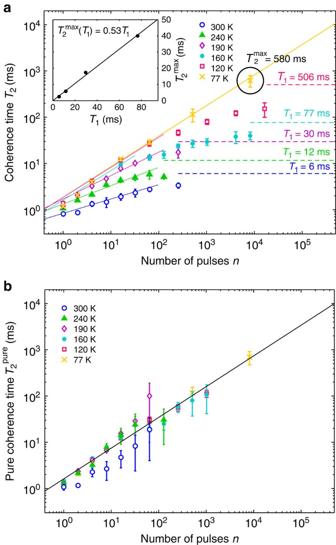Figure 2: Measured coherence time and extracted ‘pure’ coherence time for different numbers of pulses at different temperatures. (a) Measured coherence timeT2as a function of the number of pulsesnin the applied CPMG sequence, for temperatures from 77 to 300 K. Error bars indicate 1σuncertainty in the fit used to extractT2(using decoherence curves as shown inFig. 1). ForT=160 K and above, the corresponding measured longitudinal relaxation timeT1is plotted as a dashed line. The black circle indicates the longestT2=580(210) ms forn=8,192 at 77 K. Inset: scaling of the maximum coherence time as a function ofT1:. (b) NV coherence time with the phononic relaxation rate [0.53(2)T1]−1subtracted to extract the ‘pure’ spin-environment-induced decoherence, with scaling behaviour of(see text). Measured NV spin coherence decay used to determine T 2 for n -pulse CPMG sequences (coloured data points and solid line fits to data), and longitudinal spin relaxation used to determine T 1 (black data points and dashed line fits to data), at ( a ) T =300 K and ( b ) T =160 K. Full size image Coherence versus number of pulses at different temperatures Figure 2a summarizes the measured dependence of T 2 on the number of CPMG pulses n for several temperatures ranging from liquid-nitrogen temperature (77 K) to room temperature (300 K). Notably, at liquid nitrogen temperature, an 8192-pulse CPMG sequence achieved a coherence time of T 2 =580 ms, which is more than two orders of magnitude longer than previous NV T 2 measurements [6] , [10] . Accumulated pulse errors limited sequences with larger n . At T =160 K, a temperature that can be reached using thermoelectric cooling rather than cryogenic fluids, we found T 2 =40(8) ms, which is an order of magnitude longer than any previous NV T 2 measurement. Thus, combined dynamical decoupling and thermoelectric cooling provides a practical way to greatly increase the NV spin coherence time, which could benefit many applications of NV ensembles, for example, precision magnetometry [10] and rotation sensing [15] , [16] . Figure 2: Measured coherence time and extracted ‘pure’ coherence time for different numbers of pulses at different temperatures. ( a ) Measured coherence time T 2 as a function of the number of pulses n in the applied CPMG sequence, for temperatures from 77 to 300 K. Error bars indicate 1 σ uncertainty in the fit used to extract T 2 (using decoherence curves as shown in Fig. 1 ). For T =160 K and above, the corresponding measured longitudinal relaxation time T 1 is plotted as a dashed line. The black circle indicates the longest T 2 =580(210) ms for n =8,192 at 77 K. Inset: scaling of the maximum coherence time as a function of T 1 : . ( b ) NV coherence time with the phononic relaxation rate [0.53(2) T 1 ] −1 subtracted to extract the ‘pure’ spin-environment-induced decoherence, with scaling behaviour of (see text). Full size image The CPMG pulse sequence used here is quite robust against noise (for example, external magnetic field fluctuations) and pulse errors, allowing us to apply thousands of pulses. This robustness allows us to extract a near-ideal limit to the coherence time T 2 achievable with perfect pulses, although it is obtained only for one specific spin component. The other transverse spin component is more sensitive to pulse errors and has a shorter decay time, which can be improved to T 2 with more optimal pulses and symmetrized pulse sequences (such as XY). The longitudinal spin component is unaffected by these pulse errors and decays with a timescale given by T 1 . We note that the measurement scheme that we use (see Methods) allows for common-mode rejection of noise, but does not remove the effect of pulse errors. We noticed a modest reduction in signal contrast and increased noise for pulse sequences of ~10,000 pulses or more ( Fig. 3 ). The resulting reduction in signal-to-noise, together with the long integration times needed, currently prevents us from increasing the coherence time to beyond ≈0.6 s (see Methods for additional technical details). In future work, we will address these issues using various approaches, including more robust composite pulses [17] that could be better suited to manipulate an inhomogeneously broadened ensemble. This will allow the long coherence times demonstrated here to be employed for enhanced spin sensing and quantum information processing. 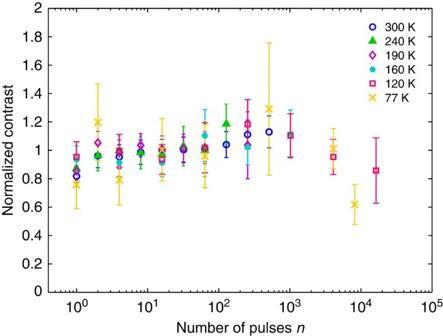Figure 3: Measured normalized signal contrastA(T,n) as a function of the number of CPMG pulsesnfor different temperaturesT. For each temperature, the contrast of the measured signalm(t) for a given pulse sequence CPMG-n(see Methods), denoted, is extracted from the fit to a stretched exponential (seeSupplementary Methods). It is then normalized against the average contrast of all pulse sequences at that temperature, denoted. Therefore, the plotted normalized contrast is given by. Figure 3: Measured normalized signal contrast A ( T , n ) as a function of the number of CPMG pulses n for different temperatures T . For each temperature, the contrast of the measured signal m ( t ) for a given pulse sequence CPMG- n (see Methods), denoted , is extracted from the fit to a stretched exponential (see Supplementary Methods ). It is then normalized against the average contrast of all pulse sequences at that temperature, denoted . Therefore, the plotted normalized contrast is given by . Full size image Relationship between maximal coherence and relaxation times The T 1 relaxation time measured for each temperature is also indicated in Fig. 2a (except for 77 K, which had T 1 >10 s). In the figure inset, we plot the maximum T 2 achieved vs. T 1 at each temperature in the interval of 160–300 K and find , which differs starkly from the previously expected T 2 limit of 2 T 1 ( [9] ). Under the assumption that spin–phonon coupling only causes spin–lattice relaxation ( T 1 ), one cannot recover the measured T 2 ≈0.5 T 1 limit, even taking into account the possibility of unequal relaxation rates between the three ground-state NV spin sublevels. This can be seen by assuming that only state-changing relaxation processes exist and, therefore, the decoherence rate between two states | a › and | b ›, , is given by [18] where is the transition rate from state | m › to state | n ›. Solving rate equations allows one to calculate the measured relaxation rate ( γ 1 =1/ T 1 ) as a function of these transition rates, and thus compare it with the decoherence rate ( γ 2 =1/ T 2 ) given by Equation (1). Through this approach one can show that for a two-level system, at temperatures ranging from zero to infinite temperature, the relation is always T 2 =2 T 1 . For three or more levels the coefficient changes, but the general statement T 2 > T 1 holds (see Supplementary Methods for further details). Therefore we conclude that in our case, as we measure T 2 < T 1 , spin–phonon coupling contributes directly and significantly to NV spin decoherence [19] . Such phonon-induced decoherence is generally relevant to any quantum system in which transitions between two levels can be driven by a two-phonon (Raman) process [11] , and could have a role in the coherence properties of many other solid-state defects. At lower temperatures, to be studied in future work, spin–spin interactions should dominate both T 1 and T 2 , and thus we expect will deviate from the ≈0.5 T 1 limit demonstrated here (see Supplementary Methods ). It is evident from Fig. 2a that the scaling of the coherence time with the number of CPMG pulses varies with temperature. In order to study the scaling behaviour of the ‘pure’ spin-environment-induced decoherence, we subtracted from the measured decoherence rate the temperature dependent phononic rate 1/[0.53(2) T 1 ] (see inset of Fig. 2a ). The corrected coherence time is plotted against the number of CPMG pulses n in Fig. 2b , exhibiting striking universal behaviour for all temperatures. We fit the corrected data to a power law scaling, and find . This value is consistent with the expected scaling power of 2/3 for a Lorentzian noise spectrum of an electronic spin bath [14] , [20] . Even though our measurements were performed on an isotopically pure sample (0.01% 13 C), we expect that similar results can be obtained for natural abundance diamond (1.1% 13 C), as the dynamical decoupling sequences we employ are also effective in suppressing dephasing caused by the nuclear spin bath [8] , [10] . However, special care must be taken in aligning the applied static magnetic field along the NV axis for natural abundance diamond since for ensembles of NVs in the presence of 13 C nuclear spins, additional decoherence is caused by variations in the effective Larmor frequency of nearby nuclear spins due to magnetic field misalignment [21] , [22] . At present we have performed measurements on one additional sample obtaining consistent results (see Methods). From this reproducibility and the ensemble nature of our experiments, we conclude that the data presents the behaviour of typical NVs, averaged over inhomogeneous broadening effects such as strain. The demonstrated improvement in coherence times for large ensembles of NV spins is directly relevant to enhanced metrology and magnetic field sensitivity [23] , [24] , which scales as ( N NV T 2 ) −1/2 , where N NV is the number of sensing NVs [2] , [10] , [25] . Thus, the hundred-fold increase in T 2 measured in this work at 77 K enables a 10-fold improvement in magnetic field sensitivity. Using samples with higher densities of NVs could further improve this sensitivity; although at high NV concentrations ( 1 p.p.b.) the coherence time may be limited by NV–NV interactions, as CPMG pulse sequences affect the NV spin and its NV spin-bath at the same time, thus cancelling the decoupling effect. Other techniques, such as WAHUHA and MREV pulse sequences [26] , [27] , may be applied to address this issue. We note that achieving long NV spin coherence times in diamond samples with high impurity concentration (~1 p.p.m.) is a crucial step towards creating non-classical states of NV ensembles. Such non-classical states could form the basis for high-sensitivity quantum metrology, potentially allowing significantly improved sensitivity and bandwidth [28] , [29] , and could also serve as a resource for quantum information protocols. To observe significant entanglement between neighbouring NV centres, their decoherence rate must be small compared with the frequency associated with their interaction. For a realistic diamond sample with [N] ~1 p.p.m. and [NV] ~10 p.p.b., coherence times larger than ~50 ms are needed for significant entanglement, which is within reach given the results presented here. For example, collective spin squeezing using one-axis squeezing techniques [30] could be created through application of pulse sequences that average-out the X , Y components of the spin–spin dipolar coupling [31] . Such pulse sequences can be straightforwardly applied in conjunction with the CPMG pulse sequences used here for extending the NV spin coherence time. In conclusion, we demonstrated more than two orders of magnitude improvement in the coherence time ( T 2 ) of ensembles of NV electronic spins in diamond compared with previous results: up to T 2 ≈0.6 s by combining dynamical decoupling control sequences with cryogenic cooling to 77 K; and ms for temperatures achievable via thermoelectric cooling (>160 K). By studying the dependence of T 2 and of the NV spin relaxation time ( T 1 ) on temperature, we identified an effective limit of T 2 ≈0.5 T 1 , which we attribute to phonon-induced decoherence. Given this limit, we expect that for low NV densities an electronic spin T 2 of a few seconds should be achievable at liquid-nitrogen temperatures ( T =77 K). The greatly extended NV spin coherence time presented in this work, which does not require an optimally chosen NV centre, could form the building block for wide-ranging applications in quantum information, sensing, and metrology in the solid-state [32] , [33] . In particular, the fact that such long coherence times can be achieved with high-density ensembles of NVs suggests that spin squeezing and highly entangled states can be created, since T 2 >NV–NV dipolar interaction time. Finally, this work could provide a key step toward realizing interaction-dominated topological quantum phases in the solid-state, as well as a large family of driven many-body quantum Hamiltonians [34] . NV structure The NV centre consists of a substitutional nitrogen atom and a vacancy occupying adjacent lattice sites in the diamond crystal ( Fig. 4a ). The electronic ground state is a spin triplet ( Fig. 4b ), in which the m s =0 and ±1 sublevels experience a ~2.87 GHz zero-field splitting. The NV centre can be rendered an effective two-level system by applying a static magnetic field to further split the m s =±1 states and addressing, for example, the m s =0 and +1 Zeeman sublevels. The NV spin can be initialized with optical excitation, detected via the state-dependent fluorescence intensity, and coherently manipulated using microwave pulse sequences [35] . 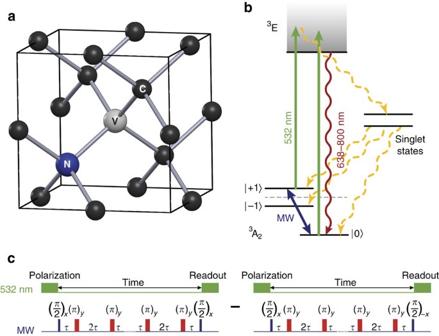Figure 4: Details of NV system and the measurement scheme and pulse sequences. (a) Lattice structure of diamond with a NV color centre. (b) Energy-level schematic of the negatively charged NV centre. (c) Measurement scheme: initialization and readout using 532 nm light, between which CPMG dynamical decoupling MW control sequences are applied. The sequence is repeated with the phase of the lastπ/2 pulse flipped (fromxto −x) for normalization (see text). Figure 4: Details of NV system and the measurement scheme and pulse sequences. ( a ) Lattice structure of diamond with a NV color centre. ( b ) Energy-level schematic of the negatively charged NV centre. ( c ) Measurement scheme: initialization and readout using 532 nm light, between which CPMG dynamical decoupling MW control sequences are applied. The sequence is repeated with the phase of the last π /2 pulse flipped (from x to − x ) for normalization (see text). Full size image Experimental set-up We performed measurements on an isotopically pure (0.01% 13 C) diamond sample (Element Six) with nitrogen density ~10 15 cm −3 and NV density ~3 × 10 12 cm −3 . The sample was mounted inside a continuous-flow cryostat (Janis ST-500) with active temperature control (Lakeshore 331). Optical excitation was done with a 532-nm laser beam focused on the diamond surface through a microscope objective (NA=0.6), and the resulting NV fluorescence was collected through the same objective and directed to a multimode fibre coupled to a single-photon counting module (Perkin-Elmer). The ~30 μm 3 detection volume contained ~100 NV centres. Microwave control pulses were delivered to the NV spins using a 70-μm diameter copper wire at the diamond surface. The experiments were performed in an unshielded environment. We measured an additional, higher density isotopically pure (0.01% 13 C) diamond sample (Element Six), with a nitrogen density ~10 17 cm −3 and NV density ~10 15 cm −3 . Owing to the higher density of the sample, the coherence times achieved were consistently lower. At T =77 K with n =4,096 pulses, we obtained a coherence time of T 2 =50(9) ms, with a scaling of the coherence time with the number of pulses of T 2 ( n )= n 0.54(1) . Pulse sequences We applied multi-pulse control sequences to decouple NV spins from the magnetic environment and thus extend the coherence time. Specifically, we used the CPMG pulse sequence [13] ( Fig. 4c ), with a varying number n of π control pulses. It has been shown previously [7] , [8] , [9] , [10] that such pulse sequences are effective in extending the coherence time T 2 of NV spins. The coherence time increases as a power law of the number of pulses T 2 n s , where the specific scaling s is determined mainly by the spin bath surrounding the NV [14] until spin-lattice relaxation begins limiting T 2 (assuming no pulse-error effects). Measurement normalization schemes The coherence measurements were performed by applying the CPMG pulse sequence with the last π /2 pulse either along the x axis or the − x axis ( Fig. 4c ). The two signals, labelled r 1 and r 2 , were then subtracted and normalized to give the measurement results m ( t )=( r 1 − r 2 )/( r 1 + r 2 ) such that common-mode noise is rejected. The final signal m ( t ) is proportional to the coherence of the NV spin, defined as the magnitude of the off-diagonal density matrix element of the m s =0,+1 two-level system C ( t )=Trace[ ρ ( t ) S x ] (with ρ ( t ) being the density matrix, and S x the transverse spin operator), at the end of the pulse sequence (before the final π /2 pulse). For a given pulse sequence (with n pulses), the NV spin coherence as a function of time was measured by varying the free precession time between pulses and thus the total sequence time. Measurements of the NV longitudinal spin relaxation followed a procedure similar to that used for the coherence measurements, with one of the two ‘common-mode’ measurements initialized to m s =0 (using an optical pumping pulse) and the other initialized to m s =+1 (using an optical pumping pulse followed by a MW π pulse). The normalized signal is proportional to the population difference between the spin states at time t , allowing measurement of the longitudinal spin relaxation and fitting to extract the T 1 relaxation time. The normalized signal contrast ( Fig. 3 ) is calculated by extracting the contrast of each decoherence curve (for example, Fig. 1 ) through a fit to a decaying stretched exponential (see Supplementary Methods ), and then normalizing this contrast by the average contrast for all pulse sequences (at a given temperature). Pulse errors The effect of pulse errors is due to amplitude and timing jitter originating in our microwave source and pulse generator. One aspect of the timing jitter is related to the pulse generator timing, which includes an output jitter of ~2 ns (negligible compared with the long duration of the pulse sequences) and a timebase accuracy of ~10 −4 . The other aspect of the timing jitter is related to the timebase of the microwave synthesizer, which has an accuracy of ~10 −10 . Timing jitter for both the pulser and the microwave synthesizer can be improved by using an external timebase. How to cite this article: Bar-Gill, N. et al . Solid-state electronic spin coherence time approaching one second. Nat. Commun. 4:1743 doi: 10.1038/ncomms2771 (2013).